Modelling Fanconi anemia pathogenesis and therapeutics using integration-free patient-derived iPSCs Fanconi anaemia (FA) is a recessive disorder characterized by genomic instability, congenital abnormalities, cancer predisposition and bone marrow (BM) failure. However, the pathogenesis of FA is not fully understood partly due to the limitations of current disease models. Here, we derive integration free-induced pluripotent stem cells (iPSCs) from an FA patient without genetic complementation and report in situ gene correction in FA–iPSCs as well as the generation of isogenic FANCA -deficient human embryonic stem cell (ESC) lines. FA cellular phenotypes are recapitulated in iPSCs/ESCs and their adult stem/progenitor cell derivatives. By using isogenic pathogenic mutation-free controls as well as cellular and genomic tools, our model serves to facilitate the discovery of novel disease features. We validate our model as a drug-screening platform by identifying several compounds that improve hematopoietic differentiation of FA–iPSCs. These compounds are also able to rescue the hematopoietic phenotype of FA patient BM cells. Fanconi Anaemia (FA) is a recessive disorder characterized by congenital abnormalities, cancer predisposition and progressive bone marrow failure (BMF) [1] , [2] . The underlying genetic defect of FA can reside in any of the sixteen FANC genes [3] , [4] , which function in a common DNA damage repair pathway. Eight FA proteins, including FANCA, form a core complex with ubiquitin E3 ligase activity. During the S phase of the cell cycle or upon DNA damage, the FA core complex monoubiquitinates the FANCD2/FANCI heterodimer, which subsequently translocates to specific nuclear foci and functions in DNA repair. Defective DNA repair in FA cells leads to G2 phase cell cycle arrest and increased cell death in response to DNA cross-linking reagents, which may contribute to the manifestation of FA disease phenotypes [1] . Patients with biallelic mutations in any of the FANC genes frequently succumb to BMF, which is the major cause of death. The mechanistic link between FA pathway deficiency and BMF remains elusive. Recent evidence in humans and mice shows that FA deficiencies lead to progressive loss of hematopoietic stem/progenitor cells and functional impairment of the repopulating ability of these cells in NOD-SCID IL2g null mice [2] , [5] , [6] , [7] . It has been suggested that a heightened p53/p21 DNA damage response induced by accumulating unrepaired DNA lesions underlies these defects, although direct evidence from patient hematopoietic stem/progenitor cells is still lacking [5] . Other than DNA repair, FA proteins also regulate proinflammatory and proapoptotic cytokine signalling. FA patient BM has been shown to overproduce tumour necrosis factor-α (TNFα) and interferon-γ (INFγ), which may suppress hematopoiesis [8] . Studying FA in primary patient cells is often impractical due to the rarity of FA, the low cellularity of patient BM and inaccessibility to certain tissues. Transformed FA cell lines have been practical surrogates, but they may not faithfully recapitulate FA disease phenotypes due to transformation-related artifacts. Although primary patient fibroblasts are useful in studying DNA damage repair in FA [9] , [10] , and while multiple mouse genetic models of FA have been developed (these models do not develop anaemia with the exception of hypomorphic Fancd1 mutation and Btbd12- deficient mouse model [11] , [12] ), understanding of stem cell defects in FA is scarce. Induced pluripotent stem cell (iPSC) technology provides the opportunity to produce various disease-relevant cell types and therefore constitutes an attractive new way to model FA [13] . However, reprogramming FA cells into iPSCs has proven to be highly inefficient [14] , [15] . We have previously shown that successful generation of FA patient-specific iPSCs (FA–iPSCs) under normoxia could be achieved if the FANCA deficiency is complemented by a lentiviral vector expressing the FANCA gene [15] . Muller et al. have since shown that reprogramming activates the FA pathway and that hypoxic conditions can facilitate lentivirus-mediated reprogramming of FA fibroblasts without genetic complementation, albeit with low efficiency [14] . More recently, Yung et al. derived FANCC deficient iPSCs under normoxia and showed increased apoptosis and reduced clonogenic potential of FANCC deficient hematopoietic progenitor cells (HPCs) derived from FA–iPSCs [16] . While these studies have improved our understanding of the role of the FA pathway in reprogramming, they also highlight challenges in establishing an iPSC-based FA model: (1) the derivation of FA–iPSCs remains highly inefficient—less than two iPSC clones established per patient fibroblast line; (2) it is still unclear whether karyotypically normal FA-deficient iPSCs can be derived without genetic complementation. Indeed, Yung et al. [16] reported a high degree of chromosomal abnormalities in FA–iPSCs (only FA-complemented iPSCs have been analysed by Muller et al. [14] ); (3) the established FA–iPSCs often fail to be maintained in culture [16] ; (4) to date, lentiviral gene complementation remains the only method of correcting FA deficiency. Because of the fact that defects in the FA pathway are associated with low efficiency in homologous recombination (HR)-dependent gene editing [17] , [18] , it is unknown whether HR-dependent gene correction approaches can be applied to FA cells. Furthermore, genetic complementation and reprogramming by viral vectors may lead to random mutagenesis and tumorigenicity [19] , which undermine the therapeutic value of the corrected cells. To avoid the issues associated with viral vectors and with the aim of improving the therapeutic potential of the FA–iPSC model, we explored the possibility of generating FA–iPSCs with episomal vectors, which are non-viral and non-integrative. To aid in studying FA pathogenesis mechanisms and developing future therapeutics, herein we report for the first time the generation of isogenic iPSC lines free of pathogenic FANCA mutation as well as FANCA −/− embryonic stem cell (ESC) lines by homologous recombination. Our model recapitulates key cellular phenotypes of FA and leads to the observation of previously unknown defects, which are rescued by targeted gene correction. Furthermore, we validate our system as a platform for drug screening, as it not only recapitulates the effects of compounds known to improve FA phenotypes, but also identifies a novel candidate that enhances hematopoietic phenotypes of FA–iPSCs/ESCs and FA BM cells. Altogether, our integration-free FA–iPSC and isogenic FA–ESC models represent a multifaceted platform to understand FA pathogenesis, discover novel therapeutic drugs and develop cell replacement therapies of FA. Generation of integration-free FA-specific iPSCs To obtain integration-free FA-specific iPSCs, we reprogrammed fibroblasts from an FA patient, who bears a biallelic truncating mutation (C295T) in the FANCA gene [20] ( Fig. 1a ), by transiently expressing five reprogramming factors (OCT4, SOX2, KLF4, LIN28, L-MYC) and p53 shRNA encoded in episomal vectors [21] , [22] . Histone deacetylase inhibitor sodium butyrate was included in the reprogramming medium to facilitate epigenetic remodelling [23] . We successfully derived FA patient-specific iPSCs under normoxia without FANCA complementation ( Fig. 1b,c ). FA fibroblasts were reprogrammed with lower efficiency (0.024% versus 0.2%) and slower kinetics (NANOG-positive colonies appeared after an average of 40 days for FA cells versus 22 days for controls) than the control fibroblasts without FANCA mutation. Despite repeated trials, we did not obtain any iPSC colony when p53 shRNA was omitted from the reprogramming cocktail even with hypoxia conditions, which are known to enhance reprogramming efficiency [24] ( Fig. 1c ). This is likely due to reprogramming barriers caused by an exacerbated p53 stress response in FA cells [14] . All FA–iPSC lines (data shown from representative clones) displayed surface makers of iPSCs ( Fig. 1d ). Importantly, we did not detect any ectopic reprogramming factor transgene or residual episomal vector sequence in five randomly selected iPSC lines (FA–iPSC#1, 2, 4, 5 and 8, Fig. 1e ). The established FA–iPSC lines displayed hallmarks of pluripotency ( Fig. 2a–c ), carried the FANCA mutation ( Fig. 1a ), were devoid of the FANCA protein ( Fig. 2d ) and demonstrated a normal karyotype at passage 13 ( Fig. 2e ). Since these fully characterized clones behaved similarly in culture, we used them interchangeably in subsequent analyses. 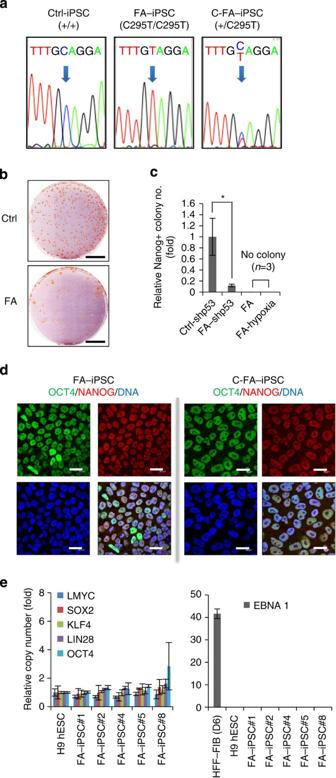Figure 1: Generation of FA-specific iPSCs. (a) DNA sequencing analysis revealed the presence of biallelic C295T point mutations inFANCAin FA–iPSCs, and the targeted correction of aFANCA-mutant allele in FA–iPSCs (C-FA–iPSCs). (b) NANOG immunostaining of control (Ctrl) and patient (FA) colonies at day 25 and day 40 of reprogramming, respectively. Scale bar, 2 cm. (c) Quantification of the number of NANOG-positive colonies at the end of reprogramming experiments. Numbers are normalized against control (mean±s.d.,n=3, *P<0.05,t-test). shp53 indicates the use of p53 shRNA in the reprogramming cocktail. In both hypoxia (5%) and normoxia conditions, there were no NANOG-positive colonies without p53 shRNA. (d) Immunofluorescence analysis of pluripotency markers OCT4 and NANOG in FA–iPSCs and C-FA–iPSCs. DNA was stained with Hoechst. Scale bar, 20 μm. (e) Copy number quantification of reprogramming factor genes (left panel) and the episomal vector element EBNA1 (right panel). H9 human ESCs were included as a negative control. Human fibroblasts (HFF-FIB) 6 days after nucleofection were included as a positive control. The average copy numbers are comparable between H9 human ESCs and five randomly selected FA–iPSCs. Data are shown as mean±s.d.n=3. Figure 1: Generation of FA-specific iPSCs. ( a ) DNA sequencing analysis revealed the presence of biallelic C295T point mutations in FANCA in FA–iPSCs, and the targeted correction of a FANCA -mutant allele in FA–iPSCs (C-FA–iPSCs). ( b ) NANOG immunostaining of control (Ctrl) and patient (FA) colonies at day 25 and day 40 of reprogramming, respectively. Scale bar, 2 cm. ( c ) Quantification of the number of NANOG-positive colonies at the end of reprogramming experiments. Numbers are normalized against control (mean±s.d., n =3, * P <0.05, t -test). shp53 indicates the use of p53 shRNA in the reprogramming cocktail. In both hypoxia (5%) and normoxia conditions, there were no NANOG-positive colonies without p53 shRNA. ( d ) Immunofluorescence analysis of pluripotency markers OCT4 and NANOG in FA–iPSCs and C-FA–iPSCs. DNA was stained with Hoechst. Scale bar, 20 μm. ( e ) Copy number quantification of reprogramming factor genes (left panel) and the episomal vector element EBNA1 (right panel). H9 human ESCs were included as a negative control. Human fibroblasts (HFF-FIB) 6 days after nucleofection were included as a positive control. The average copy numbers are comparable between H9 human ESCs and five randomly selected FA–iPSCs. Data are shown as mean±s.d. n =3. 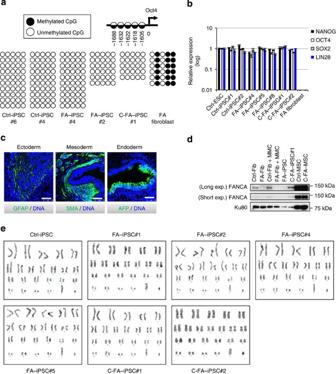Figure 2: Characterization of FA-specific iPSCs. (a) DNA methylation profile of the OCT4 promoter region in control-, FA–iPSCs and C-FA–iPSCs. A diagram showing the position of the CpG dinucleotides relative to the OCT4 transcription start site is provided. (b) RT–qPCR analysis of endogenous expression of the indicated pluripotency genes in the indicated lines. FA fibroblasts and H9 human ESCs (Ctrl-ESC) were included as negative and positive controls, respectively. Data are shown as mean±s.d.n=3. (c) Immunostaining in teratomas derived from FA–iPSCs showin vivodifferentiation towards ectodermal, mesodermal and endodermal tissues. Scale bar, 75 μm. (d) Western blotting analysis of FANCA expression in iPSCs, MSCs and fibroblasts (Fib) treated with or without MMC. Ku80 was included as a loading control. Also seeSupplementary Fig. 8. (e) Karyotyping analysis revealed normal karyotypes in all of the indicated iPSC lines. For FA–iPSC, four clones were randomly selected. C-FA–iPSC#1 and C-FA–iPSC#2 indicate FA–iPSCs corrected by HR and lentiviral vector, respectively. Full size image Figure 2: Characterization of FA-specific iPSCs. ( a ) DNA methylation profile of the OCT4 promoter region in control-, FA–iPSCs and C-FA–iPSCs. A diagram showing the position of the CpG dinucleotides relative to the OCT4 transcription start site is provided. ( b ) RT–qPCR analysis of endogenous expression of the indicated pluripotency genes in the indicated lines. FA fibroblasts and H9 human ESCs (Ctrl-ESC) were included as negative and positive controls, respectively. Data are shown as mean±s.d. n =3. ( c ) Immunostaining in teratomas derived from FA–iPSCs show in vivo differentiation towards ectodermal, mesodermal and endodermal tissues. Scale bar, 75 μm. ( d ) Western blotting analysis of FANCA expression in iPSCs, MSCs and fibroblasts (Fib) treated with or without MMC. Ku80 was included as a loading control. Also see Supplementary Fig. 8 . ( e ) Karyotyping analysis revealed normal karyotypes in all of the indicated iPSC lines. For FA–iPSC, four clones were randomly selected. C-FA–iPSC#1 and C-FA–iPSC#2 indicate FA–iPSCs corrected by HR and lentiviral vector, respectively. Full size image Characterization of FA–iPSCs FA cells are characterized by excessive G2/M arrest in the cell cycle [25] . We observed an increased G2/M cell cycle arrest in FA–iPSCs when compared with their wild-type counterparts ( Fig. 3a ). Even though FA–iPSC lines could be serially subcultured (up to passage 60 at the time of manuscript submission), they showed a decrease in clonogenicity when compared with control iPSCs ( Fig. 3b ). Monoubiquitination of FANCD2, which is indicative of a functional FA core complex that includes FANCA, was reduced in FA–iPSCs ( Fig. 3c ). In addition, FA–iPSCs failed to form FANCD2 nuclear foci upon treatment with a DNA cross-linking reagent—mitomycin C (MMC) ( Fig. 3d ). FA–iPSCs also displayed sensitivity to DNA cross-linking reagents and chromosome fragility [26] ( Fig. 3e,f ). Altogether, these observations demonstrated a defective DNA repair pathway in FA–iPSCs. 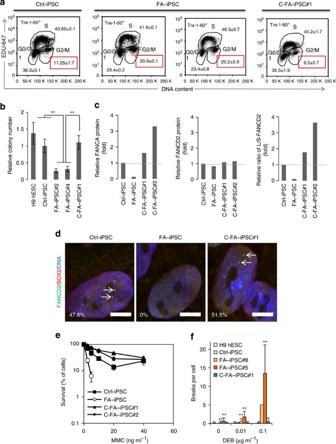Figure 3: FA-iPSCs recapitulate FA cellular defects. (a) FACS analysis of cell cycle profiles of the indicated iPSCs revealed an increased percentage of G2/M phase cells (indicated in red squares) in two randomly selected FA–iPSCs. C-FA–iPSC#1 indicates the targeted gene-correction clone. Values shown are mean±s.d. (b) An identical number of iPSCs were seeded onto MEF feeder cells in the presence of ROCK inhibitor and allowed to form small colonies. The relative iPSC colony numbers were determined 10 days later. Data are shown as mean±s.d.n=3. **P<0.01 (t-test). (c) Western blotting analysis of FANCA and FANCD2 expression in indicated iPSC lines. WRN was included as a loading control. L-FANCD2 and S-FANCD2 indicate the mono-ubiquitinated and non-modified form of FANCD2, respectively. Quantitative analysis shows that targeted correction of theFANCAgene (C-FA–iPSC#1) or lentiviral introduction of FANCA in FA–iPSCs (C-FA–iPSC#2) restored expression of FANCA protein and monoubiquitination of FANCD2. (d) Immunostaining of FANCD2 and SOX2 in the indicated iPSCs treated with 100 ng ml−1MMC for 24 h. The percentage of nuclei positive for FANCD2 foci is indicated in the bottom left corner. Scale bar, 10 μm. Arrows denote FANCD2 foci. (e) MMC sensitivity of Ctrl-iPSCs, FA–iPSCs, C-FA–iPSCs#1, and FA–iPSCs lentivirally transduced with FANCA (C-FA–iPSC#2). Data are shown as mean±s.d.n=8. (f) DEB induced chromosomal fragility test. Statistical analyses were performed by comparing Ctrl-iPSCs with other samples. Data are shown as mean±s.d.n=35 **P<0.01 (t-test). Figure 3: FA-iPSCs recapitulate FA cellular defects. ( a ) FACS analysis of cell cycle profiles of the indicated iPSCs revealed an increased percentage of G2/M phase cells (indicated in red squares) in two randomly selected FA–iPSCs. C-FA–iPSC#1 indicates the targeted gene-correction clone. Values shown are mean±s.d. ( b ) An identical number of iPSCs were seeded onto MEF feeder cells in the presence of ROCK inhibitor and allowed to form small colonies. The relative iPSC colony numbers were determined 10 days later. Data are shown as mean±s.d. n =3. ** P <0.01 ( t -test). ( c ) Western blotting analysis of FANCA and FANCD2 expression in indicated iPSC lines. WRN was included as a loading control. L-FANCD2 and S-FANCD2 indicate the mono-ubiquitinated and non-modified form of FANCD2, respectively. Quantitative analysis shows that targeted correction of the FANCA gene (C-FA–iPSC#1) or lentiviral introduction of FANCA in FA–iPSCs (C-FA–iPSC#2) restored expression of FANCA protein and monoubiquitination of FANCD2. ( d ) Immunostaining of FANCD2 and SOX2 in the indicated iPSCs treated with 100 ng ml −1 MMC for 24 h. The percentage of nuclei positive for FANCD2 foci is indicated in the bottom left corner. Scale bar, 10 μm. Arrows denote FANCD2 foci. ( e ) MMC sensitivity of Ctrl-iPSCs, FA–iPSCs, C-FA–iPSCs#1, and FA–iPSCs lentivirally transduced with FANCA (C-FA–iPSC#2). Data are shown as mean±s.d. n =8. ( f ) DEB induced chromosomal fragility test. Statistical analyses were performed by comparing Ctrl-iPSCs with other samples. Data are shown as mean±s.d. n =35 ** P <0.01 ( t -test). Full size image Targeted correction of the FANCA mutation in FA–iPSCs A major challenge in developing HR-dependent gene correction approaches in FA cells is that defects in the FA pathway are associated with inefficient HR-dependent gene editing [17] , [18] . Helper-dependent adenoviral vectors (HDAdVs) have been shown to mediate efficient gene targeting/correction via HR at various genomic loci with minimal impact on genomic integrity [21] , [27] , [28] . This non-integrative vector is devoid of the virus genome, thus minimizing cytotoxicity [29] , [30] . We performed targeted correction of the FANCA mutation in FA–iPSCs by using an HDAdV-based gene correction vector— FANCA- c-HDAdV, covering the genomic region from the promoter to intron 7 of the FANCA gene ( Fig. 4a ). Targeted gene correction was confirmed by PCR, Southern blot and sequencing analyses ( Figs 1a and 4b,c ). Further sequencing analysis confirmed that the correction was due to HR between the FANCA locus and the FANCA -c-HDAdV ( Supplementary Fig. 1A ). We next excised the integrated neomycin-resistant gene cassette using the FLP/FLPo recognition target ( FRT ) system ( Supplementary Fig. 1B ). As a complementary approach, we also generated a corrected FA–iPSC line by gene complementation using a lentiviral FANCA expression vector, similar to the one that will be used in an upcoming clinical trial [31] . These genetically corrected cells retained pluripotency and a normal karyotype ( Figs 1d and 2a,b,e ). 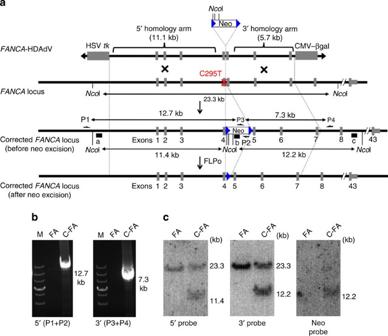Figure 4: Gene correction of FA-specific iPSCs. (a) Schematic representation of HDAdV-based correction of the C295T mutation at theFANCAlocus. The HDAd vector includes a neomycin-resistant cassette (Neo) and an HSVtkcassette to allow for positive and negative selection, respectively. Half arrows indicate primer sites for PCR (P1, P2, P3 and P4). Probes for Southern analysis are shown as black bars (a, 5′ probe;b, neo probe;c, 3′ probe). The red X indicates the mutation site in exon 4. Blue triangles indicate theFRTsite. (b) PCR analysis of FA–iPSCs (FA) and gene-corrected FA–iPSCs (C-FA) using 5′ primer pair (P1 and P2; 12.7 kb) or 3′ primer pair (P3 and P4; 7.3 kb). M, DNA ladder. (c) Southern blot analysis. The approximate molecular weights (kb) corresponding to the bands are indicated. Figure 4: Gene correction of FA-specific iPSCs. ( a ) Schematic representation of HDAdV-based correction of the C295T mutation at the FANCA locus. The HDAd vector includes a neomycin-resistant cassette (Neo) and an HSV tk cassette to allow for positive and negative selection, respectively. Half arrows indicate primer sites for PCR (P1, P2, P3 and P4). Probes for Southern analysis are shown as black bars ( a , 5′ probe; b , neo probe; c , 3′ probe). The red X indicates the mutation site in exon 4. Blue triangles indicate the FRT site. ( b ) PCR analysis of FA–iPSCs (FA) and gene-corrected FA–iPSCs (C-FA) using 5′ primer pair (P1 and P2; 12.7 kb) or 3′ primer pair (P3 and P4; 7.3 kb). M, DNA ladder. ( c ) Southern blot analysis. The approximate molecular weights (kb) corresponding to the bands are indicated. Full size image Since heterozygous carriers of FA mutations are not symptomatic [20] , we reasoned that the corrected FA–iPSCs bearing one wild-type allele might hold therapeutic potential. As expected, gene correction restored the FANCA protein expression (see C-FA–iPSC#1 in Fig. 2d ). Consistently, the cell cycle and clonogenicity defects in FA–iPSCs were also rescued by FANCA correction ( Fig. 3a,b ). FANCD2 monoubiquitination was restored by either targeted gene correction of FANCA or lentiviral delivery of the FANCA transgene (C-FA–iPSC#2) in diseased iPSCs ( Fig. 3c ). At the cellular level, gene-corrected FA–iPSCs regained the capability to form FANCD2 nuclear foci after MMC treatment ( Fig. 3d ). Consequently, MMC sensitivity and chromosomal fragility in FA–iPSCs were rescued by gene correction via HR or genetic complementation ( Fig. 3e,f ). Therefore, the FA-specific cellular defects observed in pluripotent stem cells appeared to be effectively reversed by targeted correction of the FANCA mutation. Differentiation of FA–iPSCs into HPCs A defective hematopoietic system is one of the main clinical manifestations of FA [5] , [32] . However, the pathogenesis of FA hematopoietic defects is incompletely understood. Since hematopoietic differentiation of human iPSCs is thought to mirror the developmental pattern of embryonic hematopoiesis, we reasoned that FA–iPSCs could provide a unique model for investigating FA pathogenesis during early hematopoietic commitment and specification in humans [33] . Upon directed differentiation towards the hematopoietic lineage, FA–iPSCs and in situ gene-corrected FA–iPSCs shared a common temporal pattern of HPC gene induction, suggesting that they underwent similar hematopoietic commitment and specification ( Fig. 5a ). However, when compared with control iPSCs, FA–iPSCs yielded a significantly lower percentage of HPCs ( Fig. 5b,c ), especially in the CD34 hi /CD43 lo population that has been shown to contain multipotent progenitors [34] . The fluorescence-activated cell sorting (FACS) data coincided with the lower levels of gene induction shown by quantitative PCR (qPCR) ( Fig. 5a–c ). Importantly, the deficit in generating HPCs was markedly rescued by FANCA correction ( Fig. 5b,c ). Furthermore, FA–HPCs were restricted to colony-forming unit-granulocyte macrophage (CFU-GM) and not able to generate colonies containing erythroblasts and/or megakaryocytes, whereas HPCs derived from C-FA–iPSCs gave rise to all typical hematopoietic colonies ( Fig. 5d,e ). Purified FA–HPCs displayed increased sensitivity to MMC when compared with control HPCs. Genetic correction of the FANCA mutation completely rescued this phenotype ( Fig. 5f ). 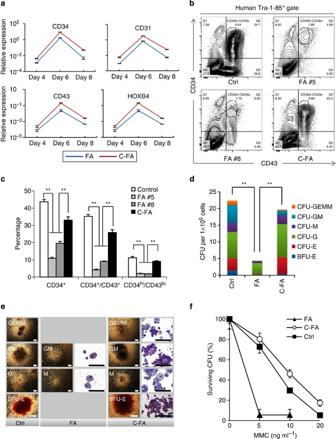Figure 5: Hematopoietic differentiation of FA–iPSCs and characterization of FA–iPSC-derived HPCs. FA–iPSCs were differentiated by using a murine OP9 stromal cell-based differentiation protocol that allows robust generation of hematopoietic cells for downstream quantitative analyses. (a) RT–qPCR analysis of the kinetics of the upregulation of hematopoietic lineage specific marker genes during hematopoietic differentiation of FA–iPSCs (FA) and FA–iPSCs corrected by HR (C-FA). Expression levels are normalized against glyceraldehyde 3-phosphate dehydrogenase. Data are shown as mean±s.e.m.n=3. (b) FACS analysis of the CD34+ and CD43+ populations 13 days after hematopoietic differentiation of control iPSCs, FA–iPSCs (#5 and #8 clones) and C-FA–iPSCs. Cells shown are in the Tra-1-85+gate, which show only human cells. Numbers represent percentages. (c) Percentage of differentiated iPSCs that are CD34+(Q1 and Q2 inb), CD34+/CD43+(Q2 inb) and CD34hi/CD43lo(small gate in Q2 inb). Error bars represent s.e.m. of three independent experiments. **P<0.01 (t-test). (d,e) Colony-forming assays of human iPSC-derived hematopoietic progenitors collected after 14 days of differentiation. Data are representative results from two independent experiments. Quantification of the indicated colony types derived from a total of 1 × 105starting differentiated cells. CFU-GEMM, colony-forming unit granulocyte/erythroid/macrophage/megakaryocyte; CFU-GM, colony-forming unit granulocyte/monocyte; CFU-M, colony-forming unit macrophage; CFU-G, colony-forming unit granulocyte; CFU-E, colony-forming unit erythroid; BFU-E, blast-forming unit erythroid.n=3. **P<0.01 (t-test). (d) Representative photos of colony morphology (left columns) and Wright staining of cytospins (right columns) of different hematopoietic colonies are shown (e). Scale bar, 300 μm. (f) MMC sensitivity of Ctrl-iPSC-, FA–iPSC- and C-FA–iPSC-derived blood lineage colonies. Data are shown as mean±s.d.n=4. Figure 5: Hematopoietic differentiation of FA–iPSCs and characterization of FA–iPSC-derived HPCs. FA–iPSCs were differentiated by using a murine OP9 stromal cell-based differentiation protocol that allows robust generation of hematopoietic cells for downstream quantitative analyses. ( a ) RT–qPCR analysis of the kinetics of the upregulation of hematopoietic lineage specific marker genes during hematopoietic differentiation of FA–iPSCs (FA) and FA–iPSCs corrected by HR (C-FA). Expression levels are normalized against glyceraldehyde 3-phosphate dehydrogenase. Data are shown as mean±s.e.m. n =3. ( b ) FACS analysis of the CD34+ and CD43+ populations 13 days after hematopoietic differentiation of control iPSCs, FA–iPSCs (#5 and #8 clones) and C-FA–iPSCs. Cells shown are in the Tra-1-85 + gate, which show only human cells. Numbers represent percentages. ( c ) Percentage of differentiated iPSCs that are CD34 + (Q1 and Q2 in b ), CD34 + /CD43 + (Q2 in b ) and CD34 hi /CD43 lo (small gate in Q2 in b ). Error bars represent s.e.m. of three independent experiments. ** P <0.01 ( t -test). ( d , e ) Colony-forming assays of human iPSC-derived hematopoietic progenitors collected after 14 days of differentiation. Data are representative results from two independent experiments. Quantification of the indicated colony types derived from a total of 1 × 10 5 starting differentiated cells. CFU-GEMM, colony-forming unit granulocyte/erythroid/macrophage/megakaryocyte; CFU-GM, colony-forming unit granulocyte/monocyte; CFU-M, colony-forming unit macrophage; CFU-G, colony-forming unit granulocyte; CFU-E, colony-forming unit erythroid; BFU-E, blast-forming unit erythroid. n =3. ** P <0.01 ( t -test). ( d ) Representative photos of colony morphology (left columns) and Wright staining of cytospins (right columns) of different hematopoietic colonies are shown ( e ). Scale bar, 300 μm. ( f ) MMC sensitivity of Ctrl-iPSC-, FA–iPSC- and C-FA–iPSC-derived blood lineage colonies. Data are shown as mean±s.d. n =4. Full size image Differentiation of FA–iPSCs into mesenchymal stem cells Mesodermal tissue defects have been reported in FA patients and mice models [35] , [36] . Given the roles of mesenchymal stem cells (MSCs) in maintaining multiple mesodermal lineages and providing a niche for normal BM hematopoietic stem cell (HSC) function [37] , we explored the possibility that human FA pathogenesis could be associated with cellular defects in MSCs. Accordingly, we differentiated control iPSCs and FA–iPSCs to MSCs ( Fig. 6a ; Supplementary Fig. 2 ). Whereas the control MSCs proliferated normally upon serial passaging, FA-iPSC-derived MSCs (FA–MSCs) failed to proliferate beyond the first three passages ( Fig. 6b ). The loss of proliferative ability was accompanied by cell senescence characteristics including enlarged and flattened cell morphology and positive staining for SA–β-galactosidase activity ( Fig. 6c ). To further support these findings, qPCR analysis was performed. When compared with control MSCs, FA–MSCs showed a robust upregulation of the cell proliferation suppressor p21, the cell senescence marker p16 and the stress sensor HO-1 as early as the first passage ( Fig. 6d ). Unlike control-iPSC-derived MSCs, which could differentiate into adipogenic, chondrogenic and osteogenic lineages in vitro , FA–MSCs failed to differentiate due to severe senescence ( Fig. 6e ). The FA–MSC-specific defects were reversed by targeted gene correction ( Figs 2d and 6b–e ). Together, these results suggest that MSC dysfunction characterized by premature senescence could be a part of the FA pathology and correction of the FANCA mutation is sufficient to normalize MSC function [35] . 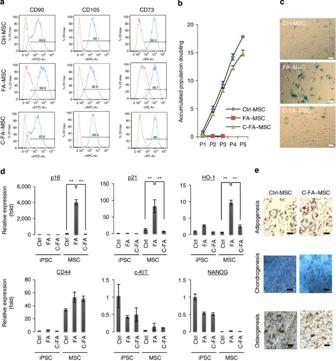Figure 6: MSCs derived from FA–iPSCs demonstrate characteristics of premature senescence. (a) FACS analyses of common MSC surface markers on MSCs differentiated from control iPSCs, FA–iPSCs and FA–iPSCs corrected by HR (C-FA–iPSCs). (b) Growth curve representing the accumulated population doubling of iPSC-derived MSCs. Data are shown as mean±s.d.n=3. (c) Representative SA–β-galactosidase staining in passage 3 MSCs derived from control-, FA–, C-FA–iPSCs. Scale bar, 100 μm. Note that senescent FA–MSCs are larger in size. (d) RT–qPCR analysis of the indicated gene transcripts in iPSCs and their MSC derivatives. Data are shown as mean±s.d.n=3. **P<0.01 (t-test). At mRNA levels, MSCs demonstrated significant upregulation of MSC-specific marker CD44 and downregulation of pluripotency marker NANOG. No significant difference was observed in NANOG and c-KIT expression between the isogenic pairs (FA–iPSCs and C-FA–iPSCs). When compared with control MSCs, FA–MSCs showed a robust upregulation of the cell proliferation suppressor p21, the cell senescence marker p16 and the stress sensor HO-1, at passage 1. (e) Control- and C-FA–iPSC-derived MSCs were induced to undergo adipogenesis, chondrogenesis and osteogenesis. Oil red, Alcian blue and von Kossa were employed for staining of adipocyte, cartilage and bone-specific markers, respectively. Scale bar, 25 μm. Figure 6: MSCs derived from FA–iPSCs demonstrate characteristics of premature senescence. ( a ) FACS analyses of common MSC surface markers on MSCs differentiated from control iPSCs, FA–iPSCs and FA–iPSCs corrected by HR (C-FA–iPSCs). ( b ) Growth curve representing the accumulated population doubling of iPSC-derived MSCs. Data are shown as mean±s.d. n =3. ( c ) Representative SA–β-galactosidase staining in passage 3 MSCs derived from control-, FA–, C-FA–iPSCs. Scale bar, 100 μm. Note that senescent FA–MSCs are larger in size. ( d ) RT–qPCR analysis of the indicated gene transcripts in iPSCs and their MSC derivatives. Data are shown as mean±s.d. n =3. ** P <0.01 ( t -test). At mRNA levels, MSCs demonstrated significant upregulation of MSC-specific marker CD44 and downregulation of pluripotency marker NANOG. No significant difference was observed in NANOG and c-KIT expression between the isogenic pairs (FA–iPSCs and C-FA–iPSCs). When compared with control MSCs, FA–MSCs showed a robust upregulation of the cell proliferation suppressor p21, the cell senescence marker p16 and the stress sensor HO-1, at passage 1. ( e ) Control- and C-FA–iPSC-derived MSCs were induced to undergo adipogenesis, chondrogenesis and osteogenesis. Oil red, Alcian blue and von Kossa were employed for staining of adipocyte, cartilage and bone-specific markers, respectively. Scale bar, 25 μm. Full size image Differentiation of FA–iPSCs into neural stem cells The spectrum of anomalies in FA extends to the nervous system; conditions such as microcephaly and mental retardation have been described among FA patients [38] , [39] , [40] . FA genes including FANCA are highly expressed in the brain of zebrafish [41] . The FA pathway has been shown to play a critical role in neural stem cell (NSC) maintenance in mice [42] . However, the aetiology of neurological manifestation of FA in humans remains elusive, partly due to a lack of appropriate experimental models. Since iPSC technology has recently been successfully used to reveal unknown neural disease phenotypes and mechanisms [43] , [44] , we next sought to study the consequence of FANCA deficiency in human neural cells. Following in vitro differentiation into NSCs ( Fig. 7a ; Supplementary Fig. 3A ), we first confirmed that FANCA expression was completely abrogated in FA–iPSCs-derived NSCs (FA–NSCs, Fig. 7b ). Upon treatment with MMC, control iPSC-derived NSCs (Ctrl-NSCs) exhibited formation of FANCD2 nuclear foci, which were completely abrogated in FA–NSCs ( Fig. 7c ). Furthermore, FA–NSCs showed an increased susceptibility to MMC-induced cell death, compared with control NSCs ( Fig. 7d ). While Ctrl-NSCs could be readily differentiated into Tuj1-positive neurons, FA–NSCs showed impaired neuronal differentiation ( Fig. 7e ; Supplementary Fig. 3B ). All these defects in FA–NSCs were rescued by targeted gene correction of FANCA ( Fig. 7b–e ; Supplementary Fig. 3B ). 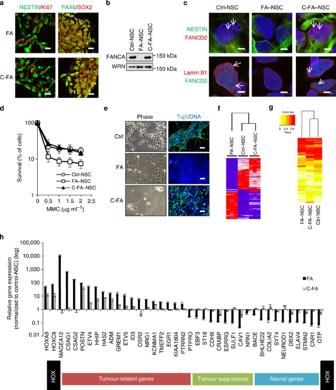Figure 7: Cellular defects and molecular signatures of NSCs derived from FA–iPSCs. (a) Immunofluorescence analysis of neural progenitor markers in FA–iPSC-derived NSCs (FA–NSCs) and C-FA–iPSC-derived NSCs (C-FA–NSCs). Scale bar, 20 μm. (b) Western blotting analysis of FANCA expression in Ctrl-NSC, FA–NSCs and C-FA–NSCs. WRN expression was included as a loading control. Also seeSupplementary Fig. 8. (c) Immunostaining of FANCD2, lamin B1 and NESTIN in the indicated NSCs treated with 100 ng ml−1MMC for 24 h. Arrows denote FANCD2 foci. Scale bar, 5 μm. (d) MMC sensitivity of indicated NSCs. Data are shown as mean±s.d.n=8. (e) Representative bright field (left panels) and Tuj1 immunofluorescence (right panels) micrographs of cultures spontaneously differentiated from Ctrl-, FA– and C-FA–NSCs. DNA was counterstained with Hoechst. Scale bar, 50 μm. (f) Hierarchical clustering analysis of genes with a minimum threefold difference in both comparisons (Ctrl-NSC versus FA–NSC; FA–NSC versus C-FA–NSC). Ninety-six percent of genes (97 out of 101) altered by the FA mutation were rescued in gene-corrected NSCs. Also seeSupplementary Data 1. (g) Heatmap and hierarchical clustering of DNA methylation levels at CpG sites in the promoter regions of the genes rescued by C-FA–NSC. Note that not every gene rescued by C-FA–NSC from gene expression analysis showed differential DNA methylation on their promoter regions. (h) RT–qPCR analysis of the expression of selected genes in passage 2 NSCs derived from Ctrl-, FA– and C-FA–iPSCs. The expression levels of genes in Ctrl-NSCs were set to one. Data are shown as mean±s.d.n=3. Gene functions are annotated below gene names. Figure 7: Cellular defects and molecular signatures of NSCs derived from FA–iPSCs. ( a ) Immunofluorescence analysis of neural progenitor markers in FA–iPSC-derived NSCs (FA–NSCs) and C-FA–iPSC-derived NSCs (C-FA–NSCs). Scale bar, 20 μm. ( b ) Western blotting analysis of FANCA expression in Ctrl-NSC, FA–NSCs and C-FA–NSCs. WRN expression was included as a loading control. Also see Supplementary Fig. 8 . ( c ) Immunostaining of FANCD2, lamin B1 and NESTIN in the indicated NSCs treated with 100 ng ml −1 MMC for 24 h. Arrows denote FANCD2 foci. Scale bar, 5 μm. ( d ) MMC sensitivity of indicated NSCs. Data are shown as mean±s.d. n =8. ( e ) Representative bright field (left panels) and Tuj1 immunofluorescence (right panels) micrographs of cultures spontaneously differentiated from Ctrl-, FA– and C-FA–NSCs. DNA was counterstained with Hoechst. Scale bar, 50 μm. ( f ) Hierarchical clustering analysis of genes with a minimum threefold difference in both comparisons (Ctrl-NSC versus FA–NSC; FA–NSC versus C-FA–NSC). Ninety-six percent of genes (97 out of 101) altered by the FA mutation were rescued in gene-corrected NSCs. Also see Supplementary Data 1 . ( g ) Heatmap and hierarchical clustering of DNA methylation levels at CpG sites in the promoter regions of the genes rescued by C-FA–NSC. Note that not every gene rescued by C-FA–NSC from gene expression analysis showed differential DNA methylation on their promoter regions. ( h ) RT–qPCR analysis of the expression of selected genes in passage 2 NSCs derived from Ctrl-, FA– and C-FA–iPSCs. The expression levels of genes in Ctrl-NSCs were set to one. Data are shown as mean±s.d. n =3. Gene functions are annotated below gene names. Full size image To elucidate the transcriptional and epigenetic alterations underlying the neurogenic defects of FA–NSCs, we conducted gene expression microarray analysis and global DNA methylation profiling. The gene expression pattern of gene-corrected NSCs (C-FA–NSCs) resembled that of Ctrl-NSCs but clustered distantly from FA–NSCs ( Fig. 7f ; Supplementary Data 1 ). Hierarchical clustering based on DNA methylation levels in the promoter region (+/−1.5 kb from transcription start site) of genes whose expression levels were rescued in C-FA–NSCs, placed C-FA–NSCs closer to Ctrl-NSCs and away from FA–NSCs ( Fig. 7g ), although this pattern was not seen at the whole-genome level ( Supplementary Fig. 3C ). This suggests that FANCA gene correction leads to specific methylation changes in a subset of promoters. Interestingly, both microarray and reverse transcriptase qPCR (RT–qPCR) analyses revealed that FA–NSCs are associated with induction of tumour-related genes, downregulation of tumour-suppressor genes, as well as downregulation of neural identity genes ( Fig. 7h ). (Epi-)genetic characterization of FA and gene-corrected cells Next, we examined whether reprogramming, gene correction and differentiation could introduce genetic instability in the FANCA -mutant genetic background. Array comparative genomic hybridization showed that C-FA–iPSCs and their derivatives did not bear additional DNA rearrangement when compared with the original FA fibroblasts, while non-corrected FA–iPSCs showed DNA rearrangements after being cultured for 40 passages ( Supplementary Fig. 4 ; Supplementary Data 2 ). We next compared the transcriptional and epigenetic status of the mutant and disease-free iPSCs at the whole-genome level. RNA-seq showed that the transcriptomes of the HDAdV-corrected (C-FA–iPSC#1) and the lentiviral vector-corrected FA–iPSCs (C-FA–iPSC#2) were similar to each other and clustered away from the two uncorrected FA–iPSC clones (FA–iPSC#5 and FA–iPSC#8, Supplementary Fig. 5A ). Similarly, whole epigenome profiling based on trimethylated H3K4 (H3K4me3) showed concordant epigenetic remodelling in the two corrected clones ( Supplementary Fig. 5B ). Together, these results reinforce the notion that the methodologies used here preserve genome stability and may provide the grounds for developing FA therapeutics. Evaluation of compounds able to reverse FA cellular defects To evaluate the utility of the FA–iPSC model in drug discovery, we screened a panel of small molecules, including a Sirt1 activator, a p38 kinase inhibitor, a synthetic androgen and an anti-inflammatory compound, for their effects on the differentiation of FA–HPCs. Resveratrol, which has been shown to partially correct hematopoietic defects in Fancd2 −/− mice [6] , did not discernibly affect HPC differentiation ( Fig. 8a,b ). However, we could not exclude the effects of resveratrol on other aspects of FA hematopoiesis. Danazol, a synthetic androgen used to treat FA, other BMF disorders and aplastic anaemia [45] , enhanced the differentiation of FA–iPSCs, C-FA–iPSCs and control iPSCs, indicating that its effects are not specific to FA. We also observed that doramapimod, a highly selective p38 MAPK inhibitor, specifically and significantly improved the derivation of CD34 + /CD43 + progenitors from FA–iPSCs ( Fig. 8a,b ). The effect of doramapimod was even more pronounced in the CD34 hi /CD43 lo population. In addition, treating purified CD34 + FA–HPCs with doramapimod enhanced CFU-GM formation, suggesting a partial rescue of the FA phenotype ( Supplementary Fig. 6A ). Our results are consistent with previous reports on the beneficial effects of p38 inhibition on FA cells [46] , [47] . Interestingly, our screen showed that tremulacin, a natural anti-inflammatory compound [48] , produced a specific and significant improvement on FA–HPC differentiation ( Fig. 8a,b ). We further asked if these compounds might exert their effects by suppressing proinflammatory and/or proapoptotic cytokine signalling in FA cells. Doramapimod and dasatinib, which have both been shown to suppress inflammatory responses [46] , [47] , significantly downregulated the expression of INFγ, TNF and interleukin 6 in FA–iPSC-derived hematopoietic cells, while danazol did not ( Fig. 8c ). Our data showed that tremulacin also potently suppressed INFγ, TNF and interleukin 6 at the transcription level ( Fig. 8c ). Interestingly, doramapimod also specifically rescued the proliferation defect of FA–MSCs but exerted no effect on the growth of gene-corrected MSCs ( Supplementary Fig. 6B ). 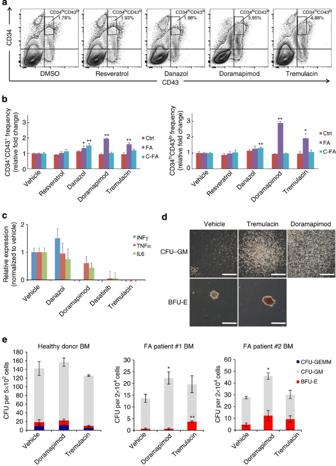Figure 8: Small-molecule screen for compounds rescuing FA hematopoietic defects. Two randomly selected clones, FA–iPSC#5 and FA–iPSC#8 (data not shown) were used in this experiment and provided consistent results. (a) FACS analysis of the CD34+and CD43+populations at day 13 of hematopoietic differentiation of FA–iPSC#5 after 1-week treatment with vehicle (DMSO), resveratrol (1 μM), danazol (50 ng ml−1), doramapimod (5 μM) and tremulacin (5 nM). (b) Quantification of percentages of FA–HPCs that are CD34+/CD43+and CD34hi/CD43loafter drug treatments indicated ina. Error bars represent s.e.m. of three independent experiments. *P<0.05 and **P<0.01 (t-test). (c) RT–qPCR quantification of expression levels of INFγ, TNFα and interleukin 6 (IL6) in differentiation cultures of FA–iPSCs treated with vehicle (DMSO), danazol (50 ng ml−1), doramapimod (5 μM), dasatinib (5 μM) and tremulacin (5 nM). Expression levels are normalized against glyceraldehyde 3-phosphate dehydrogenase. Asterisks denote expression levels below the detection limit. (d,e) Colony-forming assay of FA patient BM mononuclear cells treated with compounds. Representative photos of the morphology of different hematopoietic colonies are shown (d). Scale bar, 500 μm. (e) Quantification of the indicated colony types derived from a total of 5 × 102BM CD34+ cells and 2 × 104BM cells from healthy donors and FA patients, respectively. CFU-GEMM, colony-forming unit granulocyte/erythroid/macrophage/megakaryocyte; CFU-GM, colony-forming unit granulocyte/monocyte; BFU-E, blast-forming unit erythroid. Data are shown as mean±s.d.n=3. *P<0.05 and **P<0.01 (t-test). Figure 8: Small-molecule screen for compounds rescuing FA hematopoietic defects. Two randomly selected clones, FA–iPSC#5 and FA–iPSC#8 (data not shown) were used in this experiment and provided consistent results. ( a ) FACS analysis of the CD34 + and CD43 + populations at day 13 of hematopoietic differentiation of FA–iPSC#5 after 1-week treatment with vehicle (DMSO), resveratrol (1 μM), danazol (50 ng ml −1 ), doramapimod (5 μM) and tremulacin (5 nM). ( b ) Quantification of percentages of FA–HPCs that are CD34 + /CD43 + and CD34 hi /CD43 lo after drug treatments indicated in a . Error bars represent s.e.m. of three independent experiments. * P <0.05 and ** P <0.01 ( t -test). ( c ) RT–qPCR quantification of expression levels of INFγ, TNFα and interleukin 6 (IL6) in differentiation cultures of FA–iPSCs treated with vehicle (DMSO), danazol (50 ng ml −1 ), doramapimod (5 μM), dasatinib (5 μM) and tremulacin (5 nM). Expression levels are normalized against glyceraldehyde 3-phosphate dehydrogenase. Asterisks denote expression levels below the detection limit. ( d , e ) Colony-forming assay of FA patient BM mononuclear cells treated with compounds. Representative photos of the morphology of different hematopoietic colonies are shown ( d ). Scale bar, 500 μm. ( e ) Quantification of the indicated colony types derived from a total of 5 × 10 2 BM CD34+ cells and 2 × 10 4 BM cells from healthy donors and FA patients, respectively. CFU-GEMM, colony-forming unit granulocyte/erythroid/macrophage/megakaryocyte; CFU-GM, colony-forming unit granulocyte/monocyte; BFU-E, blast-forming unit erythroid. Data are shown as mean±s.d. n =3. * P <0.05 and ** P <0.01 ( t -test). Full size image To test if doramapimod and tremulacin could dampen the TNFα overproduction observed in FA patient cells, we utilized an FA patient-derived B-cell line that has been shown to produce TNFα constitutively [49] . Consistent with the previous data, doramapimod treatment significantly reduced secreted TNFα from patient cells ( P =0.00004, Student’s t -test [46] Supplementary Fig. 6C ), while treatment with tremulacin lead to a small yet consistent reduction of secreted TNFα when compared with treatment with the vehicle (DMSO, P =0.00117, Student’s t -test, Supplementary Fig. 6C ). Tremulacin treatment also significantly reduced TNF messenger RNA ( P =0.0123, Student’s t -test), while the effect of doramapimod did not reach statistical significance ( Supplementary Fig. 6D ). This is consistent with the fact that doramapimod acts post transcriptionally to suppress TNFα secreation [49] . These data suggest that tremulacin may function by suppressing the inflammatory response in FA cells. It is unlikely that suppression of TNFα is the sole mechanism of action of tremulacin. Future study is necessary to elucidate the pathways through which tremulacin affects hematopoietic differentiation of FA–iPSCs. The observation that FA-deficient cells overproduce proinflammatory cytokines to which they are hypersensitive suggests that aberrant cytokine signalling may underlie BM dysfunction in FA. It also underpins the hypothesis that inhibiting the action of these proinflammatory cytokines (for example, TNFα) could improve FA BM function. However, this has not been shown experimentally. Because our data show that doramapimod and tremulacin suppressed TNFα and rescued hematopoietic phenotypes of FA–HPCs, we investigated if these compounds could rescue the hematopoietic defects of FA patient BM. FA BM treated with doramapimod or tremulacin produced CFU-GMs that contained more cells than those obtained from vehicle-treated samples ( Fig. 8d ). In patient #1, erythroid colonies (burst-forming unit-erythroid or BFU-E) from tremulacin-treated samples contained mostly dark red cells, indicating high levels of haemoglobin expression, while those from vehicle-treated BM consisted of cells that were pale red or colourless ( Fig. 8d ). No difference in the apperence of BFU-Es was noted in FA patient #2. Quantification showed that doramapimod significantly increased the frequency of CFU-GM in BM of two FA patients. Tremulacin increased the mean frequency of BFU-E in both patients, although only the case in FA patient #1 was statistically significant ( Fig. 8e ). Neither doramapimod nor tremulacin had any significant effect on BM of a healthy donor ( Fig. 8e ). Generation of isogenic human ESC model of FA To independently validate the findings in our FA iPSC model, we generated three FANCA −/− H9 ESC lines (ESC–FA −/− ) by performing two rounds of transcription activator-like effector nuclease (TALEN)-mediated gene targeting ( Fig. 9a,b ). As expected, ESC–FA −/− did not express FANCA and recapitulated the cell cycle and MMC sensitivity phenotypes seen in FA–iPSCs ( Fig. 9c–e ). Following the same protocols described in the FA–iPSC model, we confirmed that ESC–FA −/− -derived HPCs, MSCs and NSCs displayed similar cellular defects as seen in the FA–iPSC model ( Fig. 9f–i ; Supplementary Fig. 7A ). We further showed that the HPC–FA −/− were not prone to apoptosis but did exhibit G2-M cell cycle arrest, which could contribute to the lower number and reduced CFU capacity of HPC–FA −/− ( Supplementary Fig. 7B,C ). Importantly, this model allowed us to independently verify the specificity of doramapimod and tremulacin in rescuing FA cellular defects ( Fig. 9j ; Supplementary Fig. 7D ). 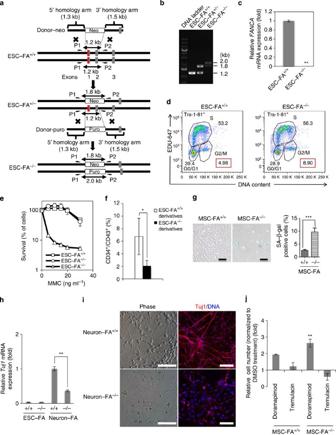Figure 9: Generation and characterization ofFANCAknockout ESCs. (a) Schematic representation of TALEN-based knockout of theFANCAgene. The donor vectors include a neomycin-resistant cassette (Neo) or a puromycin-resistant cassette (Puro). Half arrows indicate primer sites for PCR (P1 and P2). The red line indicates the TALEN target site in exon 1. Human H9 cells were used as wild-type host cells (ESC–FA+/+). The heterozygousFANCA-mutant ESC line (ESC–FA+/−) was generated by one round of gene targeting, and the biallelicFANCAknockout-mutant ESC line (ESC–FA−/−) was generated by a second round of gene targeting. (b) PCR analysis of ESC–FA+/+, ESC–FA+/−and ESC–FA−/−using P1 and P2 primer pairs shown ina. M, DNA ladder. (c) RT–PCR analysis of ESC–FA+/+and ESC–FA−/−. ESC–FA−/−did not expressFANCAmRNA. Data are shown as mean±s.d.n=3. **P<0.01 (t-test). (d) FACS analysis of cell cycle profiles of the indicated ESCs revealed an increased percentage of G2/M phase cells (indicated in red squares) inFANCAknockout cell (ESC–FA−/−). (e) MMC sensitivity of ESC–FA+/+, ESC–FA+/−and ESC–FA−/−. Data are shown as mean±s.d.n=8. (f) Percentage of differentiated ESCs that are CD34+/CD43+. Error bars represent s.e.m. of three independent experiments. *P<0.05 (t-test). (g) Representative SA–β-galactosidase staining (left panel, scale bar, 200 μm) in passage 1 MSCs derived from ESC–FA+/+and ESC–FA−/−and quantitative data (right panel). (h) RT–qPCR analysis ofTuj1in ESCs and their pan neuron derivatives. Data are shown as mean±s.d.n=3. **P<0.01 (t-test). (i) Representative bright field (left panels) and Tuj1 immunofluorescence (right panels) micrographs of cultures spontaneously differentiated from NSC–FA+/+and NSC–FA−/−. DNA was counterstained with Hoechst. Scale bar, 100 μm. (j) Quantification of accumulated doubling population of FA–MSCs with doramapimod or tremulacin treatments at passage 5. The drug effects were normalized by the number of DMSO-treated cells. Data are shown as mean±s.d.n=3. *P<0.05 (t-test). Figure 9: Generation and characterization of FANCA knockout ESCs. ( a ) Schematic representation of TALEN-based knockout of the FANCA gene. The donor vectors include a neomycin-resistant cassette (Neo) or a puromycin-resistant cassette (Puro). Half arrows indicate primer sites for PCR (P1 and P2). The red line indicates the TALEN target site in exon 1. Human H9 cells were used as wild-type host cells (ESC–FA +/+ ). The heterozygous FANCA -mutant ESC line (ESC–FA +/− ) was generated by one round of gene targeting, and the biallelic FANCA knockout-mutant ESC line (ESC–FA −/− ) was generated by a second round of gene targeting. ( b ) PCR analysis of ESC–FA +/+ , ESC–FA +/− and ESC–FA −/− using P1 and P2 primer pairs shown in a . M, DNA ladder. ( c ) RT–PCR analysis of ESC–FA +/+ and ESC–FA −/− . ESC–FA −/− did not express FANCA mRNA. Data are shown as mean±s.d. n =3. ** P <0.01 ( t -test). ( d ) FACS analysis of cell cycle profiles of the indicated ESCs revealed an increased percentage of G2/M phase cells (indicated in red squares) in FANCA knockout cell (ESC–FA −/− ). ( e ) MMC sensitivity of ESC–FA+/+, ESC–FA +/− and ESC–FA −/− . Data are shown as mean±s.d. n =8. ( f ) Percentage of differentiated ESCs that are CD34 + /CD43 + . Error bars represent s.e.m. of three independent experiments. * P <0.05 ( t -test). ( g ) Representative SA–β-galactosidase staining (left panel, scale bar, 200 μm) in passage 1 MSCs derived from ESC–FA +/+ and ESC–FA −/− and quantitative data (right panel). ( h ) RT–qPCR analysis of Tuj1 in ESCs and their pan neuron derivatives. Data are shown as mean±s.d. n =3. ** P <0.01 ( t -test). ( i ) Representative bright field (left panels) and Tuj1 immunofluorescence (right panels) micrographs of cultures spontaneously differentiated from NSC–FA +/+ and NSC–FA −/− . DNA was counterstained with Hoechst. Scale bar, 100 μm. ( j ) Quantification of accumulated doubling population of FA–MSCs with doramapimod or tremulacin treatments at passage 5. The drug effects were normalized by the number of DMSO-treated cells. Data are shown as mean±s.d. n =3. * P <0.05 ( t -test). Full size image Considering that FA pathophysiology cannot be fully recapitulated in mouse models [50] , there is a great need for human FA disease models. Here, we generated human FA-specific iPSCs without genomic integration of transgenes. In addition, we generated isogenic control iPSC lines using HDAdV-mediated targeted correction of the FANCA mutation. To the best of our knowledge, this is the first example of targeted correction of FA iPSCs. Furthermore, we verified that genome stability was preserved in C-FA–iPSCs and their differentiated progeny. We also generated isogenic FANCA −/− ESC lines by TALEN-mediated gene targeting. These isogenic ESC lines allowed us to independently validate our findings in the FA iPSC model. Our current study is limited to FA subgroup A, in which over 1,500 pathogenic mutations in the FANCA gene have been reported ( http://www.rockefeller.edu/fanconi/genes/jumpa ). The FANCA -c-HDAdV vector covers 161 (or 10%) of these mutations in FANCA . From a therapeutic point of view, more vectors are needed to correct other mutations of FANCA . Engineered nucleases, including TALEN and clustered, regularly interspaced, short palindromic repeat (CRISPR)/CAS9 nuclease and zinc-finger nuclease, could potentially be useful tools in the gene correction of FA. However, the extent of off-target mutagenesis by these methods remains controversial. Further studies are necessary to clarify whether these nuclease-based methods can be safely applied to FA. The strategy presented here can also be applied to model other subgroups of FA. Given the complexity of the FA group, these additional FA–iPSC models are necessary to cover the full spectrum of FA pathology. Many aspects of FA pathogenesis are insufficiently understood because of the scarcity of patient samples. For example, dysfunctions in MSCs and NSCs have been suggested but poorly investigated [35] , [36] , [51] . FA–iPSCs could offer unlimited research materials for unravelling yet unidentified FA phenotypes. We illustrate this point by differentiating iPSCs into three types of progenitor/stem cells, and reveal that FA pathology may entail dysfunctions in multiple progenitor/stem cell populations. FA–HPCs and FA–MSCs show similar deficiencies in maintenance and proliferation. A recent study reported that Fancg- deficient mice exhibit impaired MSC proliferation accompanied by a decreased ability to support the adhesion and engraftment of HPCs [36] . The novel MSC proliferation defect could also be associated with bone malformations in FA, as osteocytes derived from these cells are compromised in FA. We cannot exclude the possibility that the profound proliferation defects of FA–iPSC-derived MSCs may be exacerbated by extensive in vitro culture and mutations potentially accumulated during reprogramming. Nonetheless, ESC–FA −/− -derived MSCs show a consistent proliferation defect, which suggests that the MSC phenotype is mainly attributable to the FANCA deficiency. As for the neural manifestations of FA, microcephaly is a common characteristic, reaching over 90% prevalence in FANCD2 patients [38] . VACTERL (vertebral anomalies, anal atresia, cardiac defects, tracheoesophageal fistula and/or oesophageal atresia, renal & radial anomalies and limb defects) with hydrocephalus syndrome is also widespread in FANCB patients. The observed neuronal differentiation defects of FA–NSCs could contribute to these neurogenesis defects. This also supports a notion that adult neurogenesis in FA individuals may be prematurely impaired [51] . In addition, reduced survival of FA–NSCs in the presence of DNA damage reagents suggests a mechanism for ageing-dependent exhaustion of the NSC pool [42] . Furthermore, our gene expression profiling shows that FA–NSCs are associated with an induction of tumour-related genes and downregulation of tumour-suppressor genes. This may be relevant to a previous report showing that FA patients carrying the FANCD1 mutation exhibit a predisposition to develop medulloblastoma [52] . These new findings suggest an increased risk of malignant transformation in FANCA -mutated neural progenitors and allow for the identification of molecular markers of FA-associated tumour risk factors for clinical diagnosis. It should be noted that data regarding FA–NSC phenotypes are subjected to the limitations of the in vitro neuronal differentiation model. In the future, it would be of interest to study the behaviour of FA–NSCs in a transplantable in vivo model. There is an unmet need for a reliable platform allowing for the screening and evaluation of novel drug candidates for the treatment of FA. Other than its value in elucidating FA pathogenesis, the FA–iPSC/ESC model could be a useful tool for pharmacologic studies. iPSCs/ESCs can be differentiated into multiple types of hematopoietic cells in unlimited amounts. The isogenic diseased and corrected FA–iPSC and isogenic ESC lines reported here provide the most stringent and scalable screening conditions against the confounding effects that may arise due to genetic background variations. We demonstrate the usefulness of our system in drug evaluation by reproducing the beneficial effects of several compounds known to correct FA phenotypes in other FA models. Moreover, our system allowed for the discovery of a novel candidate drug for the alleviation of FA phenotypes. Although further study is needed to understand its mechanisms of action, tremulacin appears to suppress inflammatory cytokines at the transcription level. Furthermore, we show that doramapimod and tremulacin could rescue the hematopoietic defects of FA patient BM. Previous studies have raised the idea that inhibiting the action of proinflammatory cytokines could improve FA BM function [46] , [53] . Our data provide the first experimental evidence supporting this hypothesis. These results validate our iPSC-based FA model as a platform for discovering novel drugs and for studying drug mechanisms of action. Finally, we showed that our FA–iPSC/ESC model complemented by a stringent isogenic disease-free control is amenable to genome-wide interrogations of novel networks of pathogenesis pathways. In summary, the FA disease model established here represents a multifaceted practical platform for studying FA pathogenesis, for discovering novel therapeutic drugs and for the development of FA cell replacement therapies. Antibodies and plasmids Antibodies were purchased from the following companies (catalogue number and dilution for immunofluorescence or FACS). BD Biosciences: anti-human CD43-APC (560198, 1:50), anti-human CD43-FITC (555475, 1:50), anti-CD34-PE (555822, 1:50), anti-CD90-FITC (555595, 1:100), anti-CD73-PE (550257, 1:50), isotype control APC (555751, 1:50), isotype control PE (555749, 1:50), isotype control FITC (555742, 1:50); Miltenyi Biotec: anti-human CD34-APC (130-090-954, 1:50), anti-human CD34-PerCP Vio700 (130-097-915, 1:50); eBioscience: anti-CD105-APC (17-1057-42, 1:100); Biolegend: Alexa Fluor 647 anti-human Ki-67 (350509, 1:20), Alexa Fluor 647 Mouse IgG1, κ Isotype control (400130, 1:20); R&D Systems: anti-human Tra-1-85-APC (FAB3195A, 1:50); Santa Cruz Biotechnology: anti-OCT-3/4 (sc-5279, 1:100), anti-SOX2 (sc-17320, 1:100), anti-Lamin B1 (sc-6217, 1:80), anti-FANCD2 (sc-20022, 1:50), recombinant human Annexin V fluorescein reagent (NX50); Abcam: anti-NANOG (ab21624, 1:100), anti-Ki67 (ab16667, 1:1,000), anti-FANCD2 (ab2187, 1:120); Millipore: anti-NESTIN (MAB5326, 1:500), Tra-1-60 (MAB4360, 1:100); Sigma: anti-β-Tubulin III/TujI (T2200, 1:500); Covance: anti-PAX6 (PRB-278P, 1:500). pCXLE-hOCT3/4, pCXLE-hOCT3/4-shp53-F, pCXLE-hSK and pCXLE-hUL were purchased from Addgene (27076, 27077, 27078, and 27080, respectively) [22] . Lentiviral FANCA expression vector (pCCL–PGK–FANCAWp) was generated in previous study [54] . For generating FANCA knockout ESCs, two TALEN expression plasmids (TAL2416 and TAL2417) were purchased from Addgene (36817 and 36818, respectively) [55] . Cells Human FA fibroblasts (FA123) (homozygous for FANCA C295T, male, 19-year-old) were previously described [20] . The control fibroblasts (FA52) were isolated from an FA patient initially bearing compound heterogeneous FANCA mutations (Mutation 1: C 3558insG (R1187E fsX28); Mutation 2: C710-5T>C (Splicing mutation, skipping of exon 8)) [56] , which upon growth obtain spontaneous reversion of the pathological FANCA alleles in the patient. This line was used as a control for FA123 in order to exclude the non-specific effect of FA-associated profound epigenetic and genetic changes. These dermal fibroblasts were obtained after signed informed consent of the donors, the approval of the Ethics Committee and the approval of the ‘Comisión de Seguimiento y Control de la Donación de Células y Tejidos Humanos del Instituto de Salud Carlos III’ (project number: 110-90-1). H9 human ESCs were purchased from WiCell Research. Human ESCs and generated iPSC lines were cultured on Matrigel or mitotically inactivated MEF cells. A FANCC patient-derived lymphoblast cell line HSC536N is purchased from the Coriell Institute and cultured as recommended by the vendor. Human BM CD34 + cells from a healthy individual were purchased from Allcells (Alameda, CA). FA patient BM cells were isolated from two FA patients bearing FANCA mutations (Patient 1: c. 710-5T>C and c. 790C>T; Patient 2: biallelic deletions at exon 15–20). These FA patient BM samples were obtained from patients that gave informed consent. Approvals were obtained from the Ethics Committee at the G. Gaslini Hospital, Genova, Italy (protocol no. J5002; date: 24/9/2010). iPSC generation One million human fibroblasts were electroporated with pCXLE-hOCT3/4-shp53-F (or pCXLE-hOCT3/4), pCXLE-hSK and pCXLE-hUL using a Nucleofector (Lonza) [21] . Four days later, cells were re-plated onto mitotically inactivated MEF feeders in human ESC medium supplemented with 0.5 mM sodium butyrate (Sigma). After an additional 10 days, the cells were switched to human ESC medium without sodium butyrate and cultured until the colonies could be mechanically picked onto new MEF feeders. For reprogramming in hypoxia, electroporated fibroblasts were cultured in a 5% O 2 condition for 40 days. The generated FA–iPSC lines were maintained by manual picking, since enzyme-mediated passaging caused compromised cell survival. Lentiviral infection of FA–iPSCs Lentiviruses were expressed and purified according to a recently published protocol [57] . FA–iPSCs cultured on MEF feeders were incubated with 10 μM Y-27632 for 3 h and then individualized with Accumax (Innovative Cell Technologies). Cells were transduced in suspension with lentiviral FANCA expression vector in the presence of Y-27632 and 4 μg ml −1 polybrene for 1 h. After brief centrifugation to remove the residual lentivirus, the cells were seeded back on fresh MEF feeders in human ESC media containing Y-27632. After being cultured for 1 week, small iPSC colonies were manually passaged onto fresh MEF feeders and expanded as new iPSC lines. Ectopic expression of FANCA protein in different FA-iPSC lines was verified by western blotting. Bisulphite sequencing Genomic DNA from the iPSC lines was extracted with Qiagen Blood and Tissue kit. Bisulphite conversion of DNA was carried out using the Zymo EZ DNA Methylation-direct Kit (Zymo Research) following the manufacturer's recommendations. A genomic fragment of the Oct4 promoter was amplified with previously published primers using the 2 × Zymo Taq Premix per manufacturer instructions [21] , [27] . PCR products were purified by gel extraction using QIAquick columns, and subsequently cloned into the pCR2.1-TOPO vector (Invitrogen). Ten clones from each sample were sequenced with the M13 universal primer. Teratoma analysis Following injection of iPSC lines into NOD-SCID or NOD-SCID IL2Rgamma null mice (Jackson Laboratories) teratoma formation was analysed to confirm pluripotency in vivo . Briefly, mice were anaesthetized and iPSCs were injected into testis. Teratoma formation was monitored. About 10–15 weeks after injection, animals were killed. Teratomas were assessed by immunostaining. The Salk Institute Institutional Animal Care and Use Committee (IACUC) and Chinese Academy of Science Institutional Animal Care and Use Committee approved all murine experiments. Protein and nucleic acid analysis Protein quantification was performed with BCA approach (Thermo Fisher Scientific). Protein lysate was subjected to NuPAGE Novex Tris-Acetate Gel or Bis-Tris Gel (Invitrogen) and electrotransferred to a Polyvinylidene fluoride membrane (Millipore). Monoubiquitination of FANCD2 in pluripotent stem cells were determined by western blotting with anti-FANCD2 antibody [32] . Total RNA extraction and cDNA synthesis were performed with TRIzol (Invitrogen) and high capability RNA-to-cDNA Mater Mix (Invitrogen). Quantitative RT–PCR was carried out with SYBR Green PCR Master Mix (Applied Biosystems). To determine copy numbers of transgenes and endogenous genes, genomic DNA was extracted with the DNeasy Blood & Tissue Kit (Qiagen) and used as template in absolute quantification qPCR assays using the standard curve method [21] , [22] . Primer sequences are given in Supplementary Table 1 . Immunofluorescence microscopy Cells were fixed with 4% formaldehyde in phosphate-buffered saline (PBS) for 20 min at room temperature, and then permeabilized with 0.4% Triton X-100. After a blocking step with 10% fetal bovine serum (FBS) in PBS, cells were incubated with the primary antibody at 4 °C overnight, followed by incubation at room temperature with the corresponding secondary antibody for 1 h. Nuclei were counterstained with Hoechst 33342 (Invitrogen). Flow cytometry analysis For cell cycle analysis of pluripotent stem cells expressing the marker Tra-1-60 or Tra-1-81, cultures of iPSCs growing on MEFs were collected using TrypLE Express (Invitrogen). Cells were incubated with a Tra-1-60 or Tra-1-81 antibody in 1% PBS–BSA for 30 min followed by incubation with a secondary Alexa Fluor 488 anti-mouse antibody (Invitrogen) for another 30 min. After this incubation, cells were fixed in aldehyde-based fixative overnight. A Click-iT EdU flow cytometry analysis kit (Invitrogen) was used to analyse the proliferation of the Tra-1-60 or Tra-1-81-positive population of cells following manufacturer’s recommendations. For cell cycle analysis of HPCs, differentiated cells were stained with anti-human CD34-PE and anti-human CD43-FITC, fixed and permeabilized using the BD Cytofix/Cytoperm kit, stained with Alexa Fluor 647 anti-human Ki-67 and 4′,6-diamidino-2-phenylindole, and then analysed on a BD LSRFortessa cytometer. For apoptosis analysis of HPCs, differentiated cells were stained with anti-human CD34-PE, anti-human CD43-APC and Annexin V FITC, and analysed on a BD LSRFortessa cytometer. Construction and preparation of helper-dependent adenoviral vectors FANCA -c-HDAdV for gene correction was generated using a BAC clone containing the human FANCA locus (CTD-2327D14, Invitrogen), that was modified using BAC Recombineering [58] . In brief, an FRT -PGK-EM7-neo-bpA- FRT fragment was recombined into intron 4 of FANCA in the BAC clone. A total of 18.3 kb of FANCA homology, including the marker cassette, was subcloned into the HDAdV plasmid pCIHDAdGT8-4 (kindly provided by Dr Kohnosuke Mitani). The generated FANCA -c-HDAdV plasmid was linearized by PI-SceI (NEB) and then transfected into 116 cells (kindly provided by Dr Philip Ng) in the presence of helper virus AdHPBGF35 (kindly provided by Dr André M. Lieber) [59] . Crude virus extracts were serially amplified in 116 cells and then purified according to a previously described method [28] , [60] . β-gal-transducing units were determined in 293 cells to define infectious vector titres. Isolation of gene-corrected human iPSCs For generation of gene-corrected iPSCs, eleven separate experiments were performed and a total of 1.97 × 10 7 FA patient iPSCs were infected with FANCA -c-HDAdV at multiplicity of infection of 3–30 β-gal-transducing units per cell. Two to four days after infection, G418 (25–450 μg ml −1 ; Invitrogen) was added to the medium to start positive selection. After 10–13 days, 4 μM Ganciclovir (Invitrogen) in addition to G418 was added to the medium to start negative selection. After an additional 5–7 days, G418/Ganciclovir double-resistant clones were transferred to 96-well plates and expanded for further characterization. Gene-targeted clones were determined by PCR of genomic DNA from drug-resistant clones with the following primers (P1, 5′-GGAACCCACTGGTCATGTTTGCTTTTGCCCAT-3′; P2, 5′-CCCCAAAGGCCTACCCGCTTCCATTGCTCA-3′; P3, 5′-CTACCTGCCCATTCGACCACCAAGCGAAACATC-3′; P4, 5′- TACCAGGTTATAGTAGCTCAGGAATGCTAAGTCGCTCA-3′; see Fig. 3a ) using LA Taq DNA Polymerase and GC Buffer (TAKARA). Long PCR cycling included a 1 min initial denaturation at 94 °C, 14 cycles of 10 s denaturation at 98 °C and a 10 min annealing and extension at 68 °C, 21 cycles of 10 s denaturation at 98 °C and a 10 min plus 5 sec per cycle annealing and extension at 68 °C plus a final extension at 68 °C for 10 min. To determine gene-corrected clones, exon 4 of FANCA was PCR-amplified with the following primers: 5′-TTGCCCACCGTTTCTCACTTTATTGAATGCAGACC-3′ and 5′-AGGCAACCATCCCGGCTGAGAGAATACCCA-3′ with Phusion High-Fidelity DNA Polymerase (NEB). Amplicons were sequenced using an ABI 3730 sequencer (Applied Biosystems). Finally, one gene-corrected clone was generated. Excision of the neomycin-resistance cassette To efficiently remove the neomycin-resistance cassette, we generated a pCAG-Flpo-2A-puro vector, which, under control of a CAG promoter, expresses the genes for Flpo recombinase [61] , and puromycin N -acetyltransferase ( puro ). FANCA gene-corrected iPSCs cultured on Matrigel were transfected with pCAG-Flpo-2A-puro vector using FuGENE HD (Promega). Two days after transfection, puromycin (1 μg ml −1 ; Invitrogen) was added to the medium to enrich Flpo recombinase-expressing cells. Two days later, puromycin was withdrawn, and after about 10 days, cells were individualized and plated onto MEF feeder cells at a density of 300–3,000 cells per 75 cm 2 in the presence of 10 μM Y-27632 (Biomol). After 2 weeks, the emerging colonies were picked and expanded. Removal of the neomycin-resistance cassette was verified by PCR using LA Taq Hot Start Version (TAKARA) and DNA sequencing with the following primers: with the following primers: 5′-GCCCACCGTTTCTCACTTTATTGAATGCAGACCA-3′ and 5′-TGCCTCCATCCAGATCAACAGAACATTGCC-3′. Generation of FANCA gene-knockout human ESCs For generation of biallelic FA gene-knockout human ESCs, we performed two rounds of TALEN-mediated gene targeting. In brief, the donor plasmids were constructed by the combination of 1.3–1.5 kb homology arms and drug resistance cassettes (neo or puro ). For the first round of gene knockout, 1.5 × 10 7 feeder-free cultured wild-type H9 human ESCs (ESC–FA +/+ ) were dissociated by TrypLE, and resuspended in 1 ml of MEF-conditioned medium containing 10 μM ROCK inhibitor Y-27632. Cells were electroporated with 10 μg of TALEN expression plasmids each (TAL2416 and TAL2417) and 30 μg of donor vectors and were plated onto 100 mm dishes precoated with 1 × 10 6 irradiated multiple drug-resistant DR4 MEFs (ATCC). Four days after electroporation, G418 (50 μg ml −1 ) was added to the medium. After 5 days, G418 concentration was increased to 100 μg ml −1 . After 14 days, G418-resistant clones were transferred to 96-well plates and expanded for genotyping. The determined heterozygous knockout clones (ESC–FA +/− ) were used in another round of gene knockout. For this, we repeated the same steps with a puromycin-resistant donor and puromycin selection (1 μg ml −1 ) instead of a neomycin-resistant donor and G418 selection. To determine biallelic knockout clones, exon 1–2 of FANCA was PCR-amplified with the following primers (P1, 5′-TCGGCTTGGTTGGCCAGGTGGTCTCT-3′ and P2, 5′-CGCCTCGGGTGTTTTCTTAGGAAAGCTGT-3′, see Fig. 8a ) with PrimeSTAR GXL DNA Polymerase (TAKARA). Finally, three biallelic FANCA knockout clones (ESC–FA −/− ) were generated. Southern blotting Ten micrograms of genomic DNA for each sample was digested with NcoI (NEB) and subjected to 4 h at 50 V on a 0.65% agarose gel. The gel was subsequently incubated in depurination buffer (0.25 M HCl) for 15 min followed by 30 min incubation in denaturation buffer (1.5 M NaCl, 0.5 M NaOH). The DNA was then blotted overnight onto a Hybond XL (GE Healthcare) by capillary transfer in denaturation buffer. The membrane was incubated in neutralization buffer (0.5 M Tris–HCl [pH 7.4], 1.5 M NaCl) for 20 min followed by ultraviolet cross-linking. The 5′ and 3′ probes were amplified from BAC DNA (CTD-2327D14) with the following primers (5′ probe, 5′-TCCCAGAGCAGAGACAGAGGAAGCCC-3′ and 5′-CACGCCCAGCCAGGACCCAT-3′; 3′ probe, 5′-GCAGGTATCACACAAATTACAGAAGATTACCA-3′ and 5′-AGGAACATACCAGCACCTCACGAT-3′) using LA Taq Hot Start Version, following the manufacturer's protocol. The probes were labelled with dCTP [α-32P] (PerkinElmer), and Southern hybridization was performed following the standard protocol. Hematopoietic differentiation Hematopoietic differentiation efficiency and hematopoietic colony formation activity were assayed as previously described [62] with some modifications. iPSCs (passage 11) and ESCs cultured on MEF feeders in human ESC medium were manually dissociated and plated on 8-day-old overgrown OP9 feeders to start differentiation. Cells were co-cultured with the OP9 feeders for 12–14 days in OP9 differentiation medium (Alpha MEM containing 10% FBS, 100 μM monothioglycerol and 50 μg ml −1 ascorbic acid) as described [62] . Differentiated cells were dissociated with collagenase and Accutase (Innovative Cell Technologies) and subjected to flow cytometry analyses, cell sorting, qPCR analyses and clonogenic progenitor cell assays. Primer sequences for qPCR are given in Supplementary Table 1 . Clonogenic progenitor cell assay Hematopoietic clonogenic assays were performed in 35-mm low-adherent plastic dishes (Stem Cell Technologies) in triplicate using 1.1 ml per dish of MethoCult GF+H4435 semisolid medium (Stem Cell Technologies) or StemMACS human HSC–CFU complete medium with Epo (Miltenyi Biotec, 130-091-280). Colony-forming cells were scored after 15 days of incubation. Cytospins were stained with Wright stain (Millipore) according to manufacturer’s instructions. Generation and characterization of MSCs In order to guide differentiation to MSCs from iPSC (passage 11) or ESC lines, groups of 10–14 EBs were plated on Matrigel-coated six-well plates in αMEM (Invitrogen) medium with 10% FBS (Gibco), 1% penicillin/streptomycin (Gibco), 10 ng ml −1 bFGF (JPC), and 5 ng ml −1 TGFb (HumanZyme). Cells were left to differentiate for 2 weeks, until confluent fibroblast-like populations appeared. After one passage, the differentiated MSC-like cells were analysed by FACS using different antibodies related to the MSC signature. Cells were stained with antibodies against CD73, CD90 and CD105. Further differentiation towards bone, cartilage and adipose cells was performed in order to demonstrate MSC functionality. In order to evaluate the differentiation capacity to osteogenic fate, MSC lines were seeded in osteogenic media (αMEM (Invitrogen) with 10% FBS, 1% penicillin/streptomycin, 10 μM β-glycerolphosphate (Sigma), 0.2 mM ascorbate-2-phosphate (Sigma) and 0.01 mM dexamethasone (Sigma)). In the same manner, to evaluate chondrogenic differentiation, pellets of 200,000 MSCs were suspended in chondrogenic media (DMEM-high glucose (Invitrogen) with 1% penicillin/streptomycin, 10 ng ml −1 TGF-β3 (R&D Systems), 50 mg ml −1 ITS+Premix (BD), 50 μg ml −1 proline (Sigma), 50 μg ml −1 ascorbate-2-P (Sigma), and 0.1 μM dexamethasone (Sigma)). For adipogenic differentiation, once MSCs reached 95–100% confluency, expansion media was replaced with adipogenic media (αMEM with 10% FBS, 1% penicillin/streptomycin, 50 μM indomethacin (Sigma), 0.5 mM IBMX (Sigma), and 1 μM dexamethasone (Sigma)). All differentiation protocols were maintained for ~21 days. Analysis of cell differentiation was performed by histochemical staining with Oil red O (adipogenic), von Kossa (osteogenic) and Alcian blue (chondrogenic) kits (IHC World). NSC generation from iPSCs and ESCs Neural induction was performed as previously described with some modifications [63] . Induction was initiated by passaging iPSCs (passage 11) or ESCs onto MEF feeder cells at roughly 20% confluency using dispase. Neural Induction Medium 1 (NIM-1: 50% Advanced DMEM/F12 (Invitrogen), 50% neurobasal (Invitrogen), 1 × N2 (Invitrogen), 1 × B27 (Invitrogen), 2 mM GlutaMAX (Invitrogen) and 10 ng ml −1 hLIF (Millipore), 4 μM CHIR99021 (Cellagentech), 3 μM SB431542 (Cellagentech), 2 μM Dorsomorphin (Sigma), and 0.1 μM Compound E (EMD Chemicals) was used for the first 2 days. Culture medium was then switched to Neural Induction Medium 2 (NIM-2: 50% Advanced DMEM/F12, 50% Neurobasal, 1 × N2, 1 × B27, 2 mM GlutaMAX, 10 ng ml −1 hLIF, 4 μM CHIR99021, 3 μM SB431542 and 0.1 μM Compound E) and maintained for 5 days. Accumax (Innovative Cell Technologies) was used to passage cells onto Matrigel-coated plates. Cultures were subsequently maintained in Neural Stem cell Maintenance Medium containing 50% Advanced DMEM/F12, 50% Neurobasal, 1 × N2, 1 × B27, 2 mM GlutaMAX, 10 ng ml −1 hLIF, 3 μM CHIR99021 and 2 μM SB431542. Neuronal differentiation assay Ten-thousand NSCs were seeded on Matrigel-coated 35 mm wells and maintained in Neural Stem cell Maintenance Medium for 3–5 days. For spontaneous neuronal differentiation, cultures were switched to differentiation medium containing DMEM/F12, 1 × N2, 1 × B27, 400 μM dbcAMP (Sigma), 200 μM Ascorbic acid (Sigma), 10 ng ml −1 BDNF (Peprotech) and 10 ng ml −1 GDNF (Peprotech). After two days, laminin (Sigma) was added to cells to encourage differentiation. Cultures were maintained in differentiation medium for a total of 14 days, followed by immunostaining with neuronal marker Tuj1. Small-molecule pharmacologic study Resveratrol (Sigma, R5010-100MG), Danazol (Sigma, D8399-100MG), Doramapimod (BIRB 796, LC Laboratories, D-2444), Dasatinib (LC Laboratories, D-3307) and Tremulacin (Santa Cruz Biotech, sc-237233) were dissolved in DMSO and used at concentrations as indicated. At least three concentrations were tested for each drug in a pilot screen, and an optimal concentration was picked in a later confirmative study. Because early hematopoietic specification of FA–iPSCs is normal, we treated the differentiating FA–iPSC for 1 week starting on day 6 of differentiation, when the expression of HPC marker genes were at the highest levels. Drugs were added at day 6 of the iPSC hematopoietic differentiation protocol, as described above, and renewed every 2 days. At the end of the differentiation, differentiated cells were harvested and used for RNA extraction for RT–qPCR analysis of gene expression, or stained with anti-human CD34-PE, anti-human CD43-FITC and anti-human Tra-1-85-APC and subjected to flow cytometric analyses as described. For colony-forming unit assay, FA–iPSCs were differentiated as described. CD34+ cells were sorted from the differentiated cells by a BD FACSAria II cytometer. Equal number of CD34+ cells was plated in Methocult (Stem Cell Technologies, H4435) in the presence of doramapimod (5 μM) and DMSO, respectively. To examine the drug effects on MSCs, iPSC and ESC-derived MSCs were cultured in the presence of doramapimod (5 μM), tremulacin (5 nM) or DMSO in passage 0–3 for iPSC-derived or in passage 0–5 for ESC-derived MSCs. The drug effects were calculated as the number of drug-treated cells normalized to the number of DMSO-treated cells. For studying the drug effects on Fanconi patient BM cells, CFU assay was performed as described above in StemMACS human HSC–CFU complete medium with Epo in triplicate in the presence of indicated compounds. Colonies were enumerated after 2 weeks. TNFα ELISA and qRT–PCR TNFα assays were performed as described previously [46] . Briefly, 100,000 HSC536N cells were seeded per well in a 96-well plate. Cells were treated with vehicle (DMSO), doramapimod (500 nM) or tremulacin (5 nM) for 6 h. After 6-h incubation, cell culture supernatants were collected and assayed for human TNFα using the human TNFα Quantikine ELISA kit (R&D Systems). The cell pellets were used for RNA extraction using the Qiagen RNeasy kit and qRT–PCR analysis of TNF messenger RNA. Primer sequences are given in Supplementary Table 1 . Cell viability analysis To measure MMC sensitivity, 2–6 × 10 4 iPSCs, 5–7 × 10 4 ESCs or 1 × 10 5 NSCs were plated on Matrigel-coated 96-well plates (CytoOne). The following day, cells were treated with 0–40 ng ml −1 (iPSC), 0–30 ng ml −1 (ESC) or 0–2 μg ml −1 (NSCs) MMC (Biomol) for 24 h. Two days after damage, survival was assessed using CellTiter 96 AQueous One Solution Cell Proliferation Assay (Promega). To measure MMC sensitivity of HPCs, CD34 + /CD43 + HPCs were FACS sorted from differentiated FA–iPSCs, C-FA–iPSCs and Ctrl-iPSCs and cultured in a medium (Stemspan, 10 ng ml −1 IGF2, 10 ng ml −1 FGFa, 50 ng ml −1 TPO, 50 ng ml −1 Flt3L and 50 ng ml −1 SCF) containing various concentrations of MMC for 24 h before being used in CFU assays as described above. Chromosome fragility test To measure a chromosomal instability with a DNA cross-link reagent, feeder-free cultured human ESCs/iPSCs were treated with 0–0.1 μg ml −1 diepoxybutane (Sigma) for 48 h. The cells were further treated with KaryoMAX Colcemid solution (Invitrogen) at a final concentration of 20 ng ml −1 for 45 min. Staining and chromosomal fragility evaluation were described in previous study [26] . RNA-seq Reads were aligned to the reference genome (hg19, GRCh37) by using the programme tophat2 (v2.0.8b) [64] considering the read strand and the annotation data (Ensembl version 70 from iGenomes website ( http://cufflinks.cbcb.umd.edu/igenomes.html )). Alignments were then fed to the programme cuffdiff [65] to estimate the differential expression between the samples choosing the 'blind' dispersion method. The results were then analysed by using the programme cummerbund [64] to make dendrograms. ChIP-seq Reads were aligned to the reference genome (hg19, GRCh37) by using the programme bowtie2 (version 2.1.0) [66] with default parameters. Mapped reads were then investigated for the presence of enrichment against the input by using the programme MACS (version 1.4.2) [67] . Peaks with false discovery rate lower or equal to 0.05 false discovery rate were kept for the further analysis. BEDtools package [68] was used for detecting the Ensembl genes (version 70) overlapping with the detected peaks. A matrix of genes containing or not peaks for every sample was created and used to calculate the dendrogram by using R ( www.r-project.org/ ). Detection of differentially enriched peaks between samples was realized by using MAnorm tool [69] . Genome-wide DNA methylation analysis Methylation sequencing with bisulphite padlock probes was performed as previously described [70] . Briefly, genomic DNA was extracted from Ctrl-NSC, FA–NSC and C-FA–NSC using QIAamp DNA Micro Kit (Qiagen). Approximately 1,000 ng of genomic DNA was bisulphite converted with EZ-96 DNA Methylation-Lightning MagPrep kit (Zymo Research). Normalized amount of the genome-wide scale padlock probe set was annealed to 250 ng of bisulphite-converted genomic DNA, circularized, amplified and barcoded by PCR using the library-free BSPP protocol [70] . The resulting bisulphite-sequencing libraries were pooled in the same molar ratio, purified with 6% TBE PAGE gel (Invitrogen) and sequenced by Illumina HiSeq2000 sequencer (110 bp, paired-end reads). The bisulphite reads were mapped to the in silico bisulphite-converted human genome sequences (hg19) by bisREADMapper [70] . DNA methylation frequency at each CpG site with minimum 10 × depth coverage was calculated. Hierarchical clustering on genome-wide DNA methylation was performed on all CpG sites shared in all three samples. Heatmap with dendrogram was generated based on the variable CpG sites in the promoter regions (1.5 kb +/− from transcription start site) of the genes rescued by C-FA–NSC. DNA microarray and bioinformatics analysis Ctrl-, FA– and C-FA–NSC samples were prepared in biological triplicates. Total RNA of all samples was extracted using Trizol Reagent (Invitrogen) and purified by RNeasy Mini Kit (Qiagen). Affymetrix GeneChip PrimeView Human Gene Expression Arrays were performed by the Functional Genomics Core Facility at the Salk Institute for Biological Studies according to the manufacturer’s protocol (Affymetrix, Santa Clara, CA). Expression signals were scanned on Affymetrix GeneChip Scanner 3000 7G. Statistical analysis of the data was performed on the GenePattern platform from the Broad Institute ( http://www.broadinstitute.org/cancer/software/genepattern/ ). Briefly, raw CEL files were imported into GenePattern software and normalized using RMA algorithm. Gene expression probes with a minimal threefold difference in both scientific comparisons (Ctrl-NSC versus FA–NSC; FA–NSC versus C-FA–NSC) were selected for further analysis. The Hierarchical Clustering analysis was performed using the Hierarchical Clustering module of the GenePattern software. The dendrograms and the heat map of the clustered gene expression data were visualized by the Hierarchical Clustering Viewer module. Array-based genomic hybridization (aCGH) aCGH was performed to identify copy number alterations in the samples of interest (FA fibroblasts, FA–iPSCs, C-FA–iPSCs and C-FA–MSCs). We used an in-house designed microarray, based in the 8 × 60 K Agilent slide platform, composed of ~60.000 oligonucleotide probes scattered throughout the Human genome, with an average coverage of 1 probe per 30 Kb in subtelomeric and pericentromeric regions, and 1/100 Kb in the remaining euchromatic portion of the genome. The design also included the recommended set of 2.118 control probes from Agilent's catalogue. Before hybridization, DNA quality was assessed by continuous reading of optical density using a Nanodrop 2000c machine (Thermo Scientific), and DNA integrity was checked by electrophoresis and Sybr Green II (Life Technologies) staining. For each sample, 500 ng of Cy5-labelled DNA was hybridized against 500 ng of a sex-matched reference DNA Cy3-labelled. For the present study, control DNA used in the hybridization was obtained from peripheral blood lymphocytes of an anonymous donor male who consented to the use of this material for research purposes. The list of copy number variations alterations present in the control sample is indicated in Supplementary Data 2 . Labelling, hybridization, slide washing and scanning were performed following Agilent's recommended protocols (Agilent Oligonucleotide Array-Based CGH for Genomic DNA Analysis—Enzymatic Labeling for Blood Cells or Tissues, v6.0, November 2008) with minor modifications, in an ozone-free environment to prevent dye degradation. Raw data from images was extracted using Feature Extraction (Agilent, Palo Alto, CA) and detection of copy number alterations was performed using ADM-2 algorithm. Statistical analysis Results are shown as mean±s.d. Comparisons were performed with Student’s t -test. Accession codes : The RNA-seq/ChIP-seq and Methylation sequencing data sets have been deposited in NCBI Gene Expression Omnibus (GEO) under accession code GSE57828 and GSE57685 , respectively. All microarray data have been deposited in NCBI-GEO repository under accession code GSE40865 . How to cite this article : Liu, G.-H. et al. Modelling Fanconi anaemia pathogenesis and therapeutics using integration-free patient-derived iPSCs. Nat. Commun. 5:4330 doi: 10.1038/ncomms5330 (2014).